Monodisperse silicon nanocavities and photonic crystals with magnetic response in the optical region It is generally accepted that the magnetic component of light has a minor role in the light–matter interaction. The recent discovery of metamaterials has broken this traditional understanding, as both the electric and the magnetic field are key ingredients in metamaterials. The top–down technology used so far employs noble metals with large intrinsic losses. Here we report on a bottom–up approach for processing metamaterials based on suspensions of monodisperse full dielectric silicon nanocavities with a large magnetic response in the near-infrared region. Experimental results and theory show that silicon-colloid-based liquid suspensions and photonic crystals made of two-dimensional arrays of particles have strong magnetic response in the near-infrared region with small optical losses. Our findings might have important implications in the bottom–up processing of large-area low-loss metamaterials working in the near-infrared region. Although it is well known that the magnetic component of the electromagnetic field does not have an important role in the light–matter interaction [1] , it is a key ingredient for metamaterials [2] , [3] , [4] . Metamaterials are fully artificial mixtures of materials, unlike any found in nature, composed of structured building blocks (mostly metallic split-ring resonators [5] , [6] , [7] and cut-wire pairs [8] , [9] ) with strong magnetic resonance whose geometry size is much smaller than the light wavelength. The strong magnetic response of metamaterials allows fascinating new phenomena and applications, such as negative refraction [10] , perfect lenses [11] and even optical cloaking [12] . However, the high optical losses of metals limit their applications in the visible and the near-infrared regions [13] , [14] , [15] , [16] . Nowadays, top–down methods like lithography are widely used to fabricate metallic metamaterials. Complicated structures combined with high-cost equipment make large-area (bigger than one centimetre in each dimension) metallic metamaterials difficult and expensive, and three-dimensional metallic metamaterials are even more difficult to obtain [14] . Nevertheless, with the help of three-dimensional laser direct writing [17] , [18] and nanoimprint [19] technology, large-area three-dimensional chiral [17] , [18] and 75 cm 2 size fishnet [19] metamaterials were achieved. In any case, new materials and strategies are necessary for facile processing large-scale metamaterials working in the visible and near-infrared regions. To overcome those obstacles, one promising approach is to use high refractive index value dielectric particles that may also show strong magnetic and electric resonances due to the Mie resonance modes, instead of metallic structures [15] , [16] . Furthermore, one very appealing strategy is to employ the well-known bottom–up approaches of colloidal self-assembly that are extensively used for photonic crystals [20] , [21] . However, it is necessary to find metamaterial building blocks with magnetic response in the optical region of interest. Several groups have proposed silicon colloids as metamaterials building blocks in the near-infrared [22] , [23] , [24] , [25] , [26] and visible [27] , [28] , [29] , [30] , [31] , [32] regions because of their strong magnetic response corresponding to the fundamental Mie mode at wavelength values up to seven times larger than the cavity radius [22] , [23] , [24] , [25] , [26] , [27] , [28] , [29] , [30] , [31] , [32] . Theoretical results on full dielectric optical antennas [28] , [29] , magnetic type optical trapping [25] and metamaterials-related devices [22] , [23] have been published. Very recently, it has been reported about the directional scattering properties of high refractive index nanoparticles produced by simultaneous excitation and mutual interference of magnetic and electric dipole resonances inside a single high refractive index particle [33] , [34] , [35] , which is a strong evidence of the magnetic response of silicon colloids at optical frequencies. Owing to the well-defined optical resonant modes, high refractive index colloids, whose size is much smaller than the wavelength of light, behave as photonic nanocavities. So far, the fabrication of high refractive index particles concerned on different approaches as lithography [34] , chemical vapour deposition [26] and laser ablation [30] , [31] , [33] methods. However, the processing of monodisperse high refractive index nanoparticles is still a challenge, which limits the usage of high refractive index particles to true nano-optics applications. A few years ago, Korgel et al . reported on the synthesis of monodisperse hydrogenated and porous silicon colloids (a-Si:H) [36] , [37] , obtained through the decomposition of trisilane (Si 3 H 8 ) in organic solvent. Those particles have a wide variety of potential uses, including fuel cells and anode materials in lithium ion batteries. Nevertheless, because of their high porosity, a-Si:H colloids have a low refractive index value not suitable for metamaterials application. In this paper, we present, to the best of our knowledge, for the first time a method for processing large-scale monodisperse and low-loss silicon nanocavities with a magnetic response in the near-infrared region. The high refractive index of nanocavities allows us to develop liquid suspensions with a clear optical magnetic response that mimics that of the single-particle building blocks. Finally, we report on the processing and optical properties of a non-close-packed two-dimensional arrays of silicon nanocavities with a distinct magnetic response in the near-infrared region. Fabrication of monodispersed silicon colloids The method for obtaining high-refractive monodispersed submicron silicon colloids can be divided into two steps. The first step concerns synthesizing a-Si:H colloids. It is based on the decomposition of Si 3 H 8 in supercritical n -hexane at high temperature, as described elsewhere [37] (details also shown in the Methods section). The second step concerns submitting particles to a vacuum-annealing treatment to obtain high refractive index silicon colloids. X-ray diffraction and Raman spectroscopy showed that the as-synthesized colloids are made of hydrogenated amorphous silicon [37] . Two different, Si 0.75 H 0.25 and Si 0.6 H 0.4, silicon colloids were studied here. 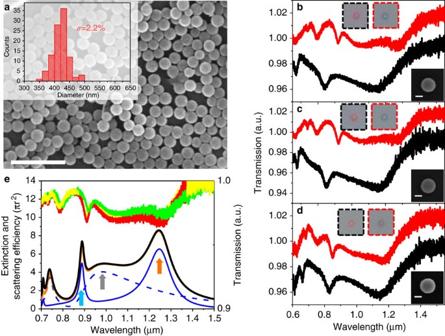Figure 1: Dispersity and optical properties of the silicon colloids. (a) SEM image (scale bar, 2,000 nm) and size distribution (inset) of Si0.75H0.25colloids. (b–d) Transmission spectra of three different single Si0.75H0.25colloids before (black line) and after (red line) an annealing process at 600, 500 and 400 °C, respectively. The optical images of the colloids before (dashed-black line-framed image) and after (dashed-red line-framed image) the annealing process are shown in the upper inset of figure. The SEM image of the corresponding annealed colloid is also shown in the lower inset of figure (scale bar, 200 nm). (e) Transmission spectra of three different colloids (yellow, red and green lines) after the annealing treatment shown in the inset. The calculated extinction (black line) and scattering (orange line) efficiencies of a single Si0.75H0.25colloid after the 600 °C annealing are also shown. The particle size and refractive index of colloids used in the calculation are 380 nm and 90% of the refractive index value of bulk silicon, respectively, which are obtained from the data shown in theSupplementary Fig. S4. The contributions of electric and magnetic resonances are presented as blue dotted and blue solid lines, respectively. The orange, grey and blue arrows correspond to the magnetic dipole, the electric dipole and the magnetic quadrupole modes based on Mie multipole expansion, respectively. Figure 1a shows the scanning electron microscope (SEM) image of spherical Si 0.75 H 0.25 430 nm large colloids with a high monodispersity, as shown in the inset of the Fig. 1a . Results on Si 0.6 H 0.4 samples are shown in the Supplementary Fig. S1 . Because of their porosity and high hydrogen content [37] , silicon colloids show different colours, red for Si 0.75 H 0.25, or bright yellow for Si 0.6 H 0.4 particles. The average diameter is around 430 nm (Si 0.75 H 0.25 ) and 460 nm (Si 0.6 H 0.4 ), respectively. In order to control the annealing process, we performed optical transmission experiments (details shown in the Methods) on several single particles. This is an important step for checking the monodispersity and the homogeneity of particles after the annealing process, to guarantee that all nanocavities show identical magnetic response. Figure 1: Dispersity and optical properties of the silicon colloids. ( a ) SEM image (scale bar, 2,000 nm) and size distribution (inset) of Si 0.75 H 0.25 colloids. ( b – d ) Transmission spectra of three different single Si 0.75 H 0.25 colloids before (black line) and after (red line) an annealing process at 600, 500 and 400 °C, respectively. The optical images of the colloids before (dashed-black line-framed image) and after (dashed-red line-framed image) the annealing process are shown in the upper inset of figure. The SEM image of the corresponding annealed colloid is also shown in the lower inset of figure (scale bar, 200 nm). ( e ) Transmission spectra of three different colloids (yellow, red and green lines) after the annealing treatment shown in the inset. The calculated extinction (black line) and scattering (orange line) efficiencies of a single Si 0.75 H 0.25 colloid after the 600 °C annealing are also shown. The particle size and refractive index of colloids used in the calculation are 380 nm and 90% of the refractive index value of bulk silicon, respectively, which are obtained from the data shown in the Supplementary Fig. S4 . The contributions of electric and magnetic resonances are presented as blue dotted and blue solid lines, respectively. The orange, grey and blue arrows correspond to the magnetic dipole, the electric dipole and the magnetic quadrupole modes based on Mie multipole expansion, respectively. Full size image Optical properties of single-particle silicon colloids Figure 1b–d shows the transmission spectra of both, the original Si 0.75 H 0.25 particles, and that after the annealing treatment at different temperatures. All the colloids are located on a glass substrate. For Si 0.75 H 0.25 colloids, 12 original a-Si:H colloids are selected arbitrarily. Three of them are shown in the Fig. 1 , and all of them are shown in the Supplementary Fig. S2 . The black curves are obtained before annealing. Because of the good monodispersity, all the selected colloids show identical optical response (black curves in Fig. 1b–d and the Supplementary Fig. S2 ). Two clear transmission dips appear in the near-infrared region. These spectral features should stem from the excitations of the optical Mie modes supported by silicon colloids. It should be mentioned that the wavelength value of the fundamental Mie mode at around 1,140 nm is five times bigger than the radius of silicon colloids. After measuring the a-Si:H colloids, they are annealed at different temperatures (300 °C to 600 °C). The red curves in Fig. 1b–d show the transmission spectra after annealing. The black and red curves in the same panel correspond to the same colloid. The transmission spectrum did not show noticeable changes after annealing at 300 °C (results shown in the Supplementary Fig. S2 ). Annealing above 400 °C, however, starts to produce a notable red shift of the transmission dips in the optical spectra. Annealing at 500 °C shifts the fundamental Mie mode (the longest wavelength optical feature) to 1,260 nm. At the same time, more transmission dips emerge. The optical images of particles also show marked differences before and after annealing (shown inset of the Fig. 1b–d ). While the as-synthesized colloids scatter a red colour [37] , this does not happen after the annealing treatment. All of this evidence indicates that the refractive index of the silicon colloids increases after annealing. These optical data are consistent with hydrogen desorption when the sample is annealed above 400 °C. For Si 0.6 H 0.4 colloids, similar results are obtained (reported in the Supplementary Fig. S3 ). The spherical colloids retain their shape after annealing, but SEM images and optical experiments show that they shrink (see inset of the Fig. 1b–d and the Supplementary Figs S2 and S3 ). Figure 1e shows the transmission spectra of three different colloids (red, green and yellow lines) after the annealing at 600 °C as well as the calculated extinction (black line) and scattering (orange line) efficiencies and the contribution of the electric (blue dashed line) and magnetic (blue solid line) resonances. From SEM images, a sphere diameter value of 380 nm was obtained, and then a fit to the Mie theory of the optical experiments yielded a refractive index value of 90% of that of bulk silicon. Here, we assumed a refractive index dispersion similar to that of bulk silicon. However, the annealed colloids may still contain some amount of porosity and hydrogen in an unknown space distribution, which could originate the observed small differences in the position of the modes between theory and experiment. More details about the size and refractive index of silicon colloids nanocavity are shown ( Supplementary Figs S4 and S5 ) and discussed in the Supplementary Notes 1 and 2 . By fitting the experimental data to the Mie theory, we can obtain information on the origin of all optical resonances. For example, the first resonant mode (the longest wavelength one) corresponds to the magnetic dipole mode, the second one corresponds to the electric dipole mode and the third one corresponds to the magnetic quadropole mode. From Fig. 1e we can conclude that, first, all annealed colloids show an identical optical signature, second, silicon colloids show a clear magnetic response corresponding to the fundamental Mie modes as the refractive index of the processed silicon colloids achieves 90% of the value of bulk silicon, third, the scattering cross section of the magnetic dipole mode is nine times bigger than the projected area, and finally, the magnetic response appears at a wavelength value six times bigger than the radius of the colloid. All in all, it indicates that the silicon colloids can be used as building blocks for developing more complex two-dimensional and three-dimensional metamaterials. Optical properties of silicon colloid suspensions We have found that silicon colloids also keep their magnetic response when dispersed in a liquid medium, allowing the processing of ‘meta-suspensions’ with a magnetic response. This is the first step for processing three-dimensional metamaterials with a bottom–up self-assembly strategy [20] , [21] . We simply ultrasonicated a liquid (toluene) dispersion of silicon colloids. As we are interested in the higher refractive index silicon colloids, only the Si 0.75 H 0.25 samples annealed at 600 °C are shown here. The optical properties of suspensions made with Si 0.75 H 0.25 particles without annealing are shown in the Supplementary Fig. S6 . 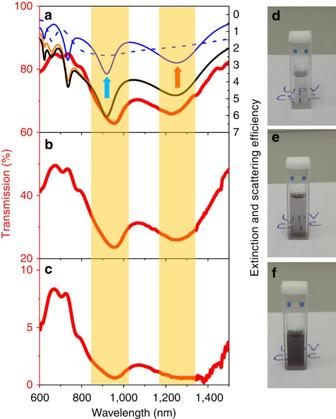Figure 2: Optical properties of annealed silicon colloids in toluene. (a) Transmission spectrum (red line) of a 600 °C annealed Si0.75H0.25colloidal suspension with a concentration of 0.005% v/v. For comparison, the calculated extinction (black line) and scattering (orange line) efficiency of a single silicon colloid immersed in toluene are also shown. The diameter and the refractive index of the silicon colloid is the same as that ofFig. 1e. The contribution of the electric (blue dash line) and the magnetic (blue solid line) resonances are also shown. The orange and blue arrows show the position of the magnetic dipole and the magnetic quadrupole modes, respectively. (b) Transmission spectrum of the same silicon colloidal suspension with a concentration of 0.01% v/v. (c) Transmission spectrum of the same silicon colloidal suspension with a concentration of 0.02% v/v. The vertical orange stripes indicate that the position of the transmission dips does not change with the solution concentration. The photos ind–fshow the measured samples. Figure 2 shows the transmission spectra and the optical images of 1-cm-thick cuvettes containing silicon colloids suspensions with different concentrations. Owing to the huge value of the scattering cross section, only a very small concentration of silicon colloids, of 0.02% v/v, blocks about 97.5% of the near-infrared light between 800 nm to 1,450 nm. These properties could be of application for near-infrared radiation blockers. Two transmission dips appear around 950 and 1,280 nm. When the concentration decreases to 0.01% v/v, those two transmission dips are more visible. At concentration values of 0.005% v/v, the sample becomes more transparent and the optical features reveal their nature. The optical transmission properties of silicon colloid suspensions are quite similar to those observed from suspensions of metallic nanoparticles [38] . However, the origin of those transmission dips is totally different. For metallic nanoparticles, the extinction phenomenon comes from the surface plasmon resonance [38] . In the silicon colloids suspension case, the optical features come from the magnetic dipole and quadrupole resonances. To prove that, Fig. 2a shows the calculated extinction (black line) and scattering (orange line) efficiencies by Mie theory of a single silicon colloid having the same values of diameter and refractive index as those detailed above, but immersed in toluene, as well as the contribution to the scattering efficiency of the magnetic modes (blue solid line) and the electric modes (blue dashed line). From this calculation, it is obvious that the transmission dip of the suspensions appearing around 1,280 nm comes from the magnetic dipole (fundamental Mie mode) and that appearing around 950 nm comes from the magnetic quadrupole mode of each colloidal nanocavity. Also, the position of the transmission dips does not change in the spectra for the three different concentrations, as indicated by the two vertical orange-coloured stripes. Therefore, we can conclude that silicon colloid meta-suspensions keep the magnetic response fingerprint of their building blocks. This happens because of the high refractive index of silicon, in comparison with the refractive index of toluene (1.496). Finally, the comparison of the extinction spectra with the scattering spectra results on a negligible absorption value of the magnetic dipole resonances. Figure 2: Optical properties of annealed silicon colloids in toluene. ( a ) Transmission spectrum (red line) of a 600 °C annealed Si 0.75 H 0.25 colloidal suspension with a concentration of 0.005% v/v. For comparison, the calculated extinction (black line) and scattering (orange line) efficiency of a single silicon colloid immersed in toluene are also shown. The diameter and the refractive index of the silicon colloid is the same as that of Fig. 1e . The contribution of the electric (blue dash line) and the magnetic (blue solid line) resonances are also shown. The orange and blue arrows show the position of the magnetic dipole and the magnetic quadrupole modes, respectively. ( b ) Transmission spectrum of the same silicon colloidal suspension with a concentration of 0.01% v/v. ( c ) Transmission spectrum of the same silicon colloidal suspension with a concentration of 0.02% v/v. The vertical orange stripes indicate that the position of the transmission dips does not change with the solution concentration. The photos in d – f show the measured samples. Full size image Optical properties of a two-dimensional photonic crystal slab In the following, we show preliminary results of a two-dimensional photonic crystal slab (2D-SiPCS) made of silicon nanocavities. 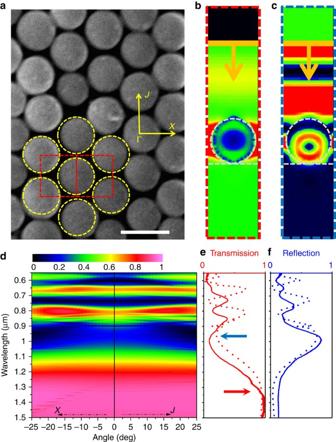Figure 3: SEM image and optical properties of a two-dimensional silicon colloids photonic crystal. (a) SEM image (scale bar, 500 nm) of a 2D-SiPCS after 600 °C annealing. The yellow dash lines show the FDTD-simulated structure being 380 nm the nanocavity diameter with a periodicity value of 430 nm. The red dash lines correspond to the simulated single cell. (b,c) Electric field distributions across the red solid line (shown ina) when the light is impinging on the sample from the top side. The field plots framed in red and blue dash lines correspond to the transmission peak (b) and dip (c) highlighted with red and blue arrows, respectively, in (e). The orange solid lines and arrows show the position of the light source in the simulation. (d) Transmittance map plot of a 2D-SiPCS as a function of the incident angle of the light and its wavelength value as obtained from the FDTD simulation. (e,f) Transmission (e) and reflection (f) spectra at Г point (zero degrees case) obtained from both the experiment (coloured solid lines) and the FDTD simulation (coloured dotted lines). Figure 3a shows the SEM image of a hexagonal lattice built by typical self-assembly methods [39] , [40] (see Methods). As the annealing process is performed on the already assembled colloidal crystal (see Methods), it shrinks the nanocavities from 430 to 380 nm (see both Methods and the Supplementary Fig. S4 ), thus resulting in a non-close-packed structure with slight disorder. Figure 3e shows the transmission (red solid line) and the reflection (blue solid line) spectra of the 2D-SiPCS at normal incidence. As the lattice parameter of the 2D-SiPCS is small, strong interactions between resonant modes of neighbours appear [23] , [27] , [28] , [29] , and the Mie theory is insufficient to describe the behaviour of 2D-SiPCS. Therefore, we have modelled the optical properties of the structure with the finite-difference time-domain (FDTD) method. The yellow dashed lines show in Fig. 3a the FDTD-simulated structure, being 380 nm the nanocavity diameter with a periodicity value of 430 nm, and the red dashed rectangle corresponds to the simulated single cell. Figure 3d shows the optical transmission contour map plot from the FDTD simulation as a function of the angle of incidence along the X and J directions of the Brillouin zone. Dashed-red (blue) curves in Fig. 3e correspond to the modelled transmission (reflection) at normal incidence of the light wave vector (zero angle value in the Fig. 3d ). FDTD calculation can roughly explain the optical features of the experiments. Dips in the transmission appear at the same wavelength values as peaks in the reflection and they correspond to the features appearing in the experiment. The discrepancies between theory and experiment can be owing either to the influence of the cavity size dispersion or to the disorder appearing in the 2D-SiPCS system. We would like to concentrate on, at first glance, the most important properties shown in Fig. 3d–f . First, at variance to the low refractive index colloidal crystals, the optical features do not shift when the angle of incidence of the light is changed ( Fig. 3d ). Second, the optical spectra of the isolated particles ( Fig. 1e ) are completely modified when they are in a close proximity, but the particle ordering does not have a key role as optical features shown in Fig. 3d does not depend on the parallel k-wavevector of the light. More experiments, which are beyond the scope of this paper, would be necessary for unveiling the role of the coupling between low-order Mie modes, especially the magnetic dipole mode, on the formation of the photonic bands. Third, in the long wavelength region above 900 nm, a near 10% transmission dip appears followed by a broad transmission peak with transmittance values near 100% ( Fig. 3e ). These transmission features can be explained by using impedance-matching arguments caused by both, the magnetic and the electric dipole interactions, [27] and it is similar to those reported very recently by Polman et al . [41] . The electric field distributions of Fig. 3b were calculated at a plane perpendicular to Fig. 3a given by the solid red line. The orange solid lines and arrows in Fig. 3b indicate the position of the light source. Inside the silicon colloids, a ring shape electric field is observed and indicates the coupling of magnetic dipole modes. The FDTD simulation in Fig. 3b shows how the wave is completely transmitted or reflected when the incident light is tuned to wavelength values corresponding to either a maximum (red arrow in Fig. 3e ) or a minimum (blue arrow in Fig. 3e ), respectively, of the transmission spectrum. In the later case, the impedance mismatch reaches maxima values, and in the former one the impedance of the 2D-SiPCS equals that of air and the transmission reaches a maximum value (near 100%). Figure 3: SEM image and optical properties of a two-dimensional silicon colloids photonic crystal. ( a ) SEM image (scale bar, 500 nm) of a 2D-SiPCS after 600 °C annealing. The yellow dash lines show the FDTD-simulated structure being 380 nm the nanocavity diameter with a periodicity value of 430 nm. The red dash lines correspond to the simulated single cell. ( b , c ) Electric field distributions across the red solid line (shown in a ) when the light is impinging on the sample from the top side. The field plots framed in red and blue dash lines correspond to the transmission peak ( b ) and dip ( c ) highlighted with red and blue arrows, respectively, in ( e ). The orange solid lines and arrows show the position of the light source in the simulation. ( d ) Transmittance map plot of a 2D-SiPCS as a function of the incident angle of the light and its wavelength value as obtained from the FDTD simulation. ( e , f ) Transmission ( e ) and reflection ( f ) spectra at Г point (zero degrees case) obtained from both the experiment (coloured solid lines) and the FDTD simulation (coloured dotted lines). Full size image The magnetic response of high refractive index colloids mostly relies on the comparison between experimental results and the Mie theory. Several works have attributed the magnetic response to the strong induced displacement current inside high refractive index particles [22] , [26] , [27] , [30] , [31] , [32] . However, it is worthy giving a complete picture of the magnetic response. The Supplementary Fig. S7 compares the magnetic response of both the silicon nanocavity and the split-ring resonator. Strong induced displacement current and magnetic field enhancement are observed in the case of the silicon nanoparticle. In the Supplementary Fig. S8 , the magnetic polarizabilities of a single silicon colloid are calculated. The calculation shows huge values for the magnetic resonances. A more detailed discussion on the relationship between the magnetic response and Mie multipole resonances of silicon colloids is shown in the Supplementary Discussion . In conclusion, submicron monodispersed silicon colloid nanocavities are fabricated and characterized. A huge magnetic response in the near-infrared region results from the high refractive index value of silicon. The high monodispersity of silicon nanocavities allows the formation of low-loss colloidal ‘meta-suspensions’ with magnetic response in the near-infrared region. Finally, we show the first experimental results of a bottom–up approach for developing a two-dimensional silicon colloidal crystal with magnetic response in the near-infrared region. These results open the door for developing new three-dimensional metamaterials through colloidal self-assembly methods. Monodispersed silicon colloids fabrication All chemicals were used as received, without further purification. Trisilane (Si 3 H 8 ; 100%) was obtained from Voltaix. (Caution: trisilane is pyrophoric and must be handled in inert atmosphere). N -hexane (95%, anhydrous) was obtained from Sigma-Aldrich. Trisilane and n -hexane were stored in a nitrogen-filled glove box. Chloroform (with 0.75% ethanol as preservative) and toluene were used as received from Fisher Scientific. a-Si:H particles were prepared by trisilane decomposition in supercritical n -hexane using a batch-scale reactor [36] , [37] . All reactions were performed at 34.5 MPa (5,000 psi). Size and hydrogen content of the particles were controlled by varying the initial trisilane concentration and reaction temperature, respectively. For these experiments, 400–500-nm-diameter particles were targeted. The reactions, targeting compositions of Si 0.75 H 0.25 and Si 0.6 H 0.4 , were performed by loading a 10 ml titanium reactor with n -hexane (5.6 and 5.8 ml, respectively) and 25 μl trisilane in a nitrogen-filled glove box. The reactors were then sealed, removed from the glove box and inserted into a preheated brass heating block at 485 and 460 °C, respectively. The temperatures were stabilized at 425 and 400 °C, respectively, and were maintained for 10 min. The reactors were then removed from the heating block and submerged in an ice bath to quench to room temperature. Here, do not exceed the maximum tolerated pressure and temperature of the reactor. The titanium reactors used for these experiments are not reliable above 69.0 MPa (10,000 psi) and 600 °C. Once the reactor cools to room temperature, the reactor is opened and the product is collected with 5 ml chloroform. At these temperatures, times and concentrations of all trisilane should be fully reacted. However, exercise caution while opening a reactor as any unreacted trisilane would ignite when exposed to air. The product is centrifuged at 8,000 r.p.m. for 5 min to precipitate the particles. The supernatant is discarded, and the particles are redispersed in toluene with light sonication and stored in ambient atmosphere. The obtained a-Si:H colloids were dried at 120 °C in an oven. The samples were then placed in a vacuum tube. The vacuum tube is directly heated to a certain temperature and maintained at that temperature for 1 h. After that, ultrasonic sound is used to disperse the silicon colloids into the toluene with a certain concentration. In the self-assembly process, Si 0.75 H 0.25 colloids, 430 nm large, are used for colloidal ordering [39] , [40] . The fabrication process of the structure is as follows. Toluene suspension of monodisperse Si 0.75 H 0.25 colloidal particles (0.02% v/v) was injected into a cell formed by two quartz plates separated by a U-shaped spacer. After drying it in air, a highly ordered monolayer array of silicon colloids was obtained. In order to remove the hydrogen from the silicon nanocavities, and also increase the refractive index value of particles, a further annealing process at 600 °C was performed. It shrinks particles from 430 to 380 nm, this leading to a non-close-packed structure. Optical measurement and the theory calculation For single silicon colloid measurements, the silicon colloids are put on a glass substrate. This glass substrate was then placed on a sample holder of a home-made confocal microscope, which allowed measuring both the transmitted and the reflected light. The unpolarized incident light is focused on the silicon colloid by a microscope objective (× 20). The light impinges from the glass substrate side onto the silicon colloid. The transmitted and reflected signals are collected and analysed by means of a spectrometer and a liquid nitrogen-refrigerated InGaAs linear array. For the silicon colloids suspensions measurements, the quartz cuvettes containing the suspensions are directly located at the entrance of the spectrometer. The cuvettes are made of quartz and the length of the light path through the cuvettes is 1 cm. For 2D-SiPCS measurements, the method is similar as that of the single silicon colloid measurements, but with a larger aperture size on the confocal plane. In the Mie theory calculations, the refractive index of toluene was considered as a constant parameter with a value of 1.496. The refractive index of pure silicon was obtained from ref. 42 . We modified the existing code [43] to calculate the extinction and scattering efficiency of single silicon colloid. The FDTD simulation is performed with the commercial software, FDTD Solutions 7.5 (Lumerical, 2011). How to cite this article: Shi, L. et al . Monodisperse silicon nanocavities and photonic crystals with magnetic response in the optical region. Nat. Commun. 4:1904 doi: 10.1038/ncomms2934 (2013).